Regulated delivery of molecular cargo to invasive tumour-derived microvesicles Cells release multiple, distinct forms of extracellular vesicles including structures known as microvesicles, which are known to alter the extracellular environment. Despite growing understanding of microvesicle biogenesis, function and contents, mechanisms regulating cargo delivery and enrichment remain largely unknown. Here we demonstrate that in amoeboid-like invasive tumour cell lines, the v-SNARE, VAMP3, regulates delivery of microvesicle cargo such as the membrane-type 1 matrix metalloprotease (MT1-MMP) to shedding microvesicles. MT1-MMP delivery to nascent microvesicles depends on the association of VAMP3 with the tetraspanin CD9 and facilitates the maintenance of amoeboid cell invasion. VAMP3-shRNA expression depletes shed vesicles of MT1-MMP and decreases cell invasiveness when embedded in cross-linked collagen matrices. Finally, we describe functionally similar microvesicles isolated from bodily fluids of ovarian cancer patients. Together these studies demonstrate the importance of microvesicle cargo sorting in matrix degradation and disease progression. Multiple cell types, including tumour cells, have been documented to shed extracellular vesicles—membrane enclosed structures released from the cell during both physiologic and disease states [1] , [2] . Unlike exosomes, which are released into the extracellular space from multivesicular bodies, shed microvesicles are formed by a direct, outward budding and pinching event, although the mechanisms underlying their biogenesis and release into the extracellular environment are only beginning to be understood [2] , [3] . Microvesicles are heterogeneous in both size and content. They range from ∼ 200 nm to a few micrometres in diameter and their cargo content varies based on both the cell type from which they originate and through the onset or progression of disease states [1] . Vesicles derived from tumour cells that fit these latter criteria have been referred to as tumour-derived microvesicles (TMVs) and oncosomes [1] , [4] , [5] . A concept emerging from recent research, the aberrant release of microvesicles is now thought to correlate with the onset and progression of many disease states, including multiple cancers, and microvesicle contents are known to change and their numbers to increase as disease worsens. In ovarian cancer, for example, the amount and proteolytic content of shed microvesicles was found to correlate with invasiveness [6] . Similarly, ascites from stage VI disease was shown to contain significantly more microvesicles than that collected from stage I disease [7] . Studies have also shown an increase in microvesicle content in the serum of gastric cancer patients and, importantly, differences in microvesicle content between patients with active head and neck squamous cell carcinoma and those in remission [8] , [9] . These disease-associated changes, coupled with the identification of shed microvesicles in bodily fluids, has heightened interest in their clinical potential. Growing understanding of the contents of TMVs and their ability to transfer bioactive molecules including lipids, proteins and functional nucleic acids to recipient cells in the extracellular microenvironment [10] , [11] , [12] has led to a host of research into their roles in the formation and progression of disease states. Shed microvesicles have been postulated to function in modulating immune responses [13] , [14] , mechanisms to resist chemotherapeutics [15] , [16] , eliciting signalling responses in surrounding cells [17] , horizontal transfer of cargo constituents [10] , [11] , paracrine signalling [18] , [19] and conditioning the tumour microenvironment [20] . The presence of proteases, such as membrane-type 1 matrix metalloprotease (MT1-MMP), in TMVs is supportive of their role in facilitating cell invasion of the extracellular matrix (ECM) [4] , [21] . With increasing understanding of TMV cargo contents, attention is shifting towards understanding the molecular regulators of intracellular traffic responsible for the sorting, delivery and enrichment of microvesicle cargo. Intracellular vesicular traffic is regulated in large part by soluble N -ethylmaleimide-sensitive factor attachment protein receptor (SNARE) proteins. The distinct localization of individual members of the SNARE family suggests that they participate in specific intracellular trafficking routes [22] , [23] , [24] . It is the combination of vesicular (v-SNARE) and target (t-SNARE) proteins that make up the core machinery necessary for intracellular membrane fusion and specified cargo delivery [24] , [25] . There is growing evidence that several SNARE proteins are involved in the traffic of MMPs. Vesicle-associated membrane protein (VAMP) 7, VAMP3 and syntaxin-4 have all been shown to participate in the intracellular movement of MT1-MMP [26] , [27] , [28] . Studies also suggest that the regulation of intracellular trafficking of MMPs is critical for the sustained ECM remodelling necessary for tumour cell invasion [28] , [29] . Here we show that in rounded, invasive tumour cell lines, VAMP3 regulates the delivery of microvesicle cargo such as MT1-MMP, to regions of high plasma membrane blebbing, regions from which TMVs are often released. Blocking protease delivery to TMVs significantly compromises movement through cross-linked collagen matrices, documenting the importance of TMVs in matrix degradation. Furthermore, we demonstrate that TMVs showing structural and functional similarity to those described above, can be isolated from peripheral body fluids of ovarian cancer patients. These studies, which provide new insight into TMV cargo sorting and their role in cancer invasion, underscore the need to better understand the complex motile behaviour of tumour cells. VAMP3 and MT1-MMP co-traffic in amoeboid cells Tumour cell invasion is a heterogeneous and adaptive process, wherein tumour cells interchangeably adopt either rounded, bleb-associated amoeboid morphologies or elongated, flattened mesenchymal-like morphologies, similar to those previously documented in migrating tumour cells [30] , [31] . We observed a striking correlation between the characteristic amoeboid phenotype and TMV formation in the invasive melanoma cell line, LOX, wherein TMVs pinch and release from regions of active surface blebbing into the extracellular space ( Fig. 1a and Supplementary Movies 1 and 2 ). Previous studies examining the cargo content of these vesicles found that VAMP3, but not VAMP7, was included in shed TMVs [4] . These studies, together with published research linking VAMP3 to the surface expression of MT1-MMP, led us to test the hypothesis that VAMP3 directs cargo to regions of surface blebbing and into nascent microvesicles [26] . To this end, we made use of live-cell imaging to track VAMP3-GFP and MT1-MMP-mCherry in LOX cells. In rounded, highly blebbing cells, we identified a pool of MT1-MMP-mCherry on VAMP3-GFP-positive intracellular vesicles ( Fig. 1b , arrows). These vesicles traffic towards the cell surface ( Fig. 1c , arrow), migrating into newly formed surface blebs ( Fig. 1d and Supplementary Movie 3 ). In contrast, elongated and flattened cells show reduced levels of VAMP3 and MT1-MMP co-localization ( Fig. 1e ). Similar results were obtained when MT1-MMP and vSNARE association was examined in prostate (PC-3) and colorectal (SW480) adenocarcinoma cell lines ( Supplementary Fig. 1a,b ). Notably, we do not observe any reduction in total VAMP3 or a significant difference in VAMP3 distribution, when cells adopt a mesenchymal-like morphology ( Supplementary Fig. 1c,d ). Instead, in mesenchymal-like cells, MT1-MMP localized to large perinuclear puncta where it resided within VAMP7 rosettes ( Fig. 1e,f and Supplementary Fig. 1a,b ). These structures, identified previously [28] , appeared predominantly along the ventral surface of the cell. In support of these observations, measurement of Pearson’s coefficient indicates that more rounded cells show greater co-distribution of MT1-MMP and VAMP3 ( Fig. 1g , upper), than flat, more elongated cells ( Fig. 1g , lower). To quantify these differences we measured the bleb index, ((blebs per second)/(cell perimeter)), which allowed uniform analysis unbiased by cell size or shape. Analysis of Pearson’s coefficient versus bleb index reveals a positive correlation between VAMP3/MT1-MMP co-localization and amoeboid or round morphology ( Fig. 1h ). Together, these experiments demonstrate that it is not an overall shift in VAMP3 localization that is responsible for directing protease cargo to sites of TMV formation, rather, as cells adopt an amoeboid morphology, the association between VAMP3 and MT1-MMP is increased. 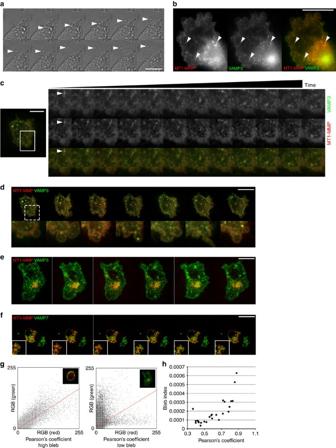Figure 1: VAMP3 and MT1-MMP co-traffic to sites of active membrane blebbing. (a) TMVs are shed from areas of high blebbing activity. Sequential frames captured during imaging of unlabelled cells plated on gelatin-coated dish. Movie frames acquired 1.5 s apart. Vesicles shed from regions of membrane blebbing (arrow). Scale bar, 20 μm. LOX cells alone or co-transfected with VAMP3-GFP and MT1-MMP-mCherry, or VAMP7-GFP and MT1-MMP-mCherry, were plated on unlabelled gelatin. Cells were visualized using phase-contrast or live-cell spinning disk confocal microscopy. (b) VAMP3-GTP and MT1-MMP-mCherry co-localize on intracellular vesicles (arrows) in amoeboid cells. Scale bar, 25 μm. (c) Small, highly mobile vesicles (arrow) containing MT1-MMP and VAMP3 travel outward from the vicinity of larger vesicular structures in an anterograde manner. Individual frames captured fromSupplementary Movie 3were captured 1.5 s apart, total time 18 s. Scale bar, 25 μm. (d) VAMP3-MT1-MMP intracellular vesicles traffic into newly formed membrane blebs. This montage is composed of stills fromSupplementary Movie 1, to highlight trafficking into membrane blebs. Scale bar, 25 μm. (e) LOX cells with flattened, mesenchymal morphology exhibit less co-localization between VAMP3 and MT1-MMP. Sequential frames∼40 s apart. Scale bar, 25 μm. (f) A pool of MT1-MMP localizes to the centre of VAMP7 rosettes. Sequential frames∼40 s apart. Scale bar, 25 μm. (g) LOX cells that have adopted an amoeboid morphology when plated on gelatin show a high level of co-localization between VAMP3 and MT1-MMP as measured by the Pearson’s coefficient (upper), while cells that adopt a flattened, mesenchymal morphology show demonstrably less co-localization between VAMP3 and MT1-MMP (lower). Images are representative. (h) Increasing bleb index* in LOX cells correlates with an increase in the co-localization between VAMP3 and MT1-MMP as measured by the Pearson’s coefficient.n=30 randomly selected cells. *Bleb index=blebs per second/cell perimeter. Figure 1: VAMP3 and MT1-MMP co-traffic to sites of active membrane blebbing. ( a ) TMVs are shed from areas of high blebbing activity. Sequential frames captured during imaging of unlabelled cells plated on gelatin-coated dish. Movie frames acquired 1.5 s apart. Vesicles shed from regions of membrane blebbing (arrow). Scale bar, 20 μm. LOX cells alone or co-transfected with VAMP3-GFP and MT1-MMP-mCherry, or VAMP7-GFP and MT1-MMP-mCherry, were plated on unlabelled gelatin. Cells were visualized using phase-contrast or live-cell spinning disk confocal microscopy. ( b ) VAMP3-GTP and MT1-MMP-mCherry co-localize on intracellular vesicles (arrows) in amoeboid cells. Scale bar, 25 μm. ( c ) Small, highly mobile vesicles (arrow) containing MT1-MMP and VAMP3 travel outward from the vicinity of larger vesicular structures in an anterograde manner. Individual frames captured from Supplementary Movie 3 were captured 1.5 s apart, total time 18 s. Scale bar, 25 μm. ( d ) VAMP3-MT1-MMP intracellular vesicles traffic into newly formed membrane blebs. This montage is composed of stills from Supplementary Movie 1 , to highlight trafficking into membrane blebs. Scale bar, 25 μm. ( e ) LOX cells with flattened, mesenchymal morphology exhibit less co-localization between VAMP3 and MT1-MMP. Sequential frames ∼ 40 s apart. Scale bar, 25 μm. ( f ) A pool of MT1-MMP localizes to the centre of VAMP7 rosettes. Sequential frames ∼ 40 s apart. Scale bar, 25 μm. ( g ) LOX cells that have adopted an amoeboid morphology when plated on gelatin show a high level of co-localization between VAMP3 and MT1-MMP as measured by the Pearson’s coefficient (upper), while cells that adopt a flattened, mesenchymal morphology show demonstrably less co-localization between VAMP3 and MT1-MMP (lower). Images are representative. ( h ) Increasing bleb index* in LOX cells correlates with an increase in the co-localization between VAMP3 and MT1-MMP as measured by the Pearson’s coefficient. n =30 randomly selected cells. *Bleb index=blebs per second/cell perimeter. Full size image VAMP3-shRNA reduces TMV and amoeboid cell-invasive capacity With results showing VAMP3 and MT1-MMP co-trafficking to sites of active surface blebbing, we focused these investigations on the requirement for VAMP3 in the delivery of MT1-MMP to shed TMVs. To this end, we used short hairpin RNA (shRNA) to knock down endogenous VAMP3 ( Supplementary Fig. 2a–c ). The shRNA plasmid contains a red fluorescent protein (RFP) reporter allowing tracking of TMVs released specifically from knockdown cells. To examine their invasive capacity, TMVs were isolated from VAMP3 knockdown or scrambled shRNA (control) cells, plated onto fluorescein isothiocyanate (FITC)-gelatin and allowed to degrade overnight ( Fig. 2a,b ). VAMP3 knockdown resulted in >70% reduction in microvesicle-mediated matrix degradation ( Fig. 2a,c ). Isolated TMVs shed from control cells contain MT1-MMP ( Fig. 2d , left) while those from VAMP3-depleted cells contained no detectable protease ( Fig. 2d , right). This reduction in MT1-MMP was confirmed by western blotting of microvesicle lysate ( Fig. 2e and Supplementary Fig. 2c ). Of note, although there was a reduction in MT1-MMP, we found no appreciable difference in other known microvesicle cargo including β 1 -integrin and major histocompatibility complex-I ( Fig. 2e and Supplementary Fig. 3 ), suggesting that VAMP3 knockdown does not significantly change the amount of TMVs released. Endogenous MT1-MMP was seen on intracellular puncta contained within budding TMVs in control cells ( Fig. 2f , upper), whereas the protease was absent in VAMP3-knockdown cells ( Fig. 2f , lower). Similar results documenting decreased TMV-associated MT1-MMP on VAMP3 depletion were obtained using prostate cancer cell line, PC-3 ( Supplementary Fig. 4 ). Thus, VAMP3 knockdown perturbs MT1-MMP trafficking and delivery to TMVs. 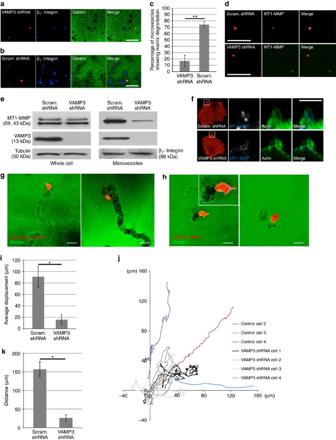Figure 2: VAMP3 knockdown disrupts trafficking and delivery of MT1-MMP and altersin vitroinvasive capacity. TMVs were isolated from LOX cells expressing VAMP3 shRNA (a) or scrambled shRNA (b). TMVs were plated on FITC-gelatin-coated coverslips and allowed to degrade substrate. Slides were fixed and stained as indicated, to show vesicle-associated matrix degradation (dark areas). Scale bar, 10 μm. TMV-associated matrix degradation quantified inc. Data presented as mean±1 s.d.;n=120 per condition across 3 independent experiments;P<0.02 determined by Student’st-test. (d) TMVs from VAMP3- or scrambled-shRNA cells were stained to examine endogenous MT1-MMP. Scale bar, 5 μm. (e) TMVs were isolated from VAMP3- or scrambled-shRNA-electroporated LOX cells, lysed and equal protein (determined by BCA) separated by SDS–PAGE, blotted and probed as indicated. Immunoblots are representative of at least three independent experiments. (f) VAMP3-shRNA- or scrambled-shRNA-transfected LOX cells were plated on unlabelled gelatin substrate. Cells were fixed and stained to identify endogenous MT1-MMP. Cells carrying scrambled shRNA show intracellular MT1-MMP identifiable in surface blebs. This staining and the presence of MT1-MMP in surface blebs are absent in VAMP3-shRNA cells. Scale bar, 5 μm. Scrambled-shRNA- (g) or VAMP3-shRNA- (h) transfected LOX cells were plated on FITC-conjugated gelatin-coated coverslips. Cells were fixed and stained as indicated, to examine the matrix degradation. Higher-magnification image of VAMP3-shRNA invasion in inset. (i) Linear displacement of the cell’s centre of mass at timet=0 and at timet=14 h. Results from a minimum of 15 cells per condition from 3 independent experiments. Data presented as mean±1 s.d.;P<0.01 determined by Studentsttest. (j) The approximate centre of mass in scrambled-shRNA- or VAMP3-shRNA-transfected cells embedded in PurCol collagen matrix was tracked over time by live-cell imaging. Positions plotted relative to the origin (timet=0). (k) Linear displacement of invading cells was quantified over 14 h. Results represent at least 15 cells per condition over independent experiments. Data presented as mean±1 s.d.;P<0.01 determined by Studentsttest. Figure 2: VAMP3 knockdown disrupts trafficking and delivery of MT1-MMP and alters in vitro invasive capacity. TMVs were isolated from LOX cells expressing VAMP3 shRNA ( a ) or scrambled shRNA ( b ). TMVs were plated on FITC-gelatin-coated coverslips and allowed to degrade substrate. Slides were fixed and stained as indicated, to show vesicle-associated matrix degradation (dark areas). Scale bar, 10 μm. TMV-associated matrix degradation quantified in c . Data presented as mean±1 s.d. ; n =120 per condition across 3 independent experiments; P <0.02 determined by Student’s t -test. ( d ) TMVs from VAMP3- or scrambled-shRNA cells were stained to examine endogenous MT1-MMP. Scale bar, 5 μm. ( e ) TMVs were isolated from VAMP3- or scrambled-shRNA-electroporated LOX cells, lysed and equal protein (determined by BCA) separated by SDS–PAGE, blotted and probed as indicated. Immunoblots are representative of at least three independent experiments. ( f ) VAMP3-shRNA- or scrambled-shRNA-transfected LOX cells were plated on unlabelled gelatin substrate. Cells were fixed and stained to identify endogenous MT1-MMP. Cells carrying scrambled shRNA show intracellular MT1-MMP identifiable in surface blebs. This staining and the presence of MT1-MMP in surface blebs are absent in VAMP3-shRNA cells. Scale bar, 5 μm. Scrambled-shRNA- ( g ) or VAMP3-shRNA- ( h ) transfected LOX cells were plated on FITC-conjugated gelatin-coated coverslips. Cells were fixed and stained as indicated, to examine the matrix degradation. Higher-magnification image of VAMP3-shRNA invasion in inset. ( i ) Linear displacement of the cell’s centre of mass at time t =0 and at time t =14 h. Results from a minimum of 15 cells per condition from 3 independent experiments. Data presented as mean±1 s.d. ; P <0.01 determined by Students t test. ( j ) The approximate centre of mass in scrambled-shRNA- or VAMP3-shRNA-transfected cells embedded in PurCol collagen matrix was tracked over time by live-cell imaging. Positions plotted relative to the origin (time t =0). ( k ) Linear displacement of invading cells was quantified over 14 h. Results represent at least 15 cells per condition over independent experiments. Data presented as mean±1 s.d. ; P <0.01 determined by Students t test. Full size image We evaluated the invasive capacity of VAMP3-depleted cells using confocal microscopy. On overnight incubation on deformable gelatin, rounded cells appear to invade with some directionality, leaving a trail of degraded matrix in their wake and covering an average of 90.8 μm ( Fig. 2g,i and Supplementary Fig. 2d,e ). In contrast, the cells expressing VAMP3 shRNA formed voids within the matrix and were displaced only 15.9 μm on average ( Fig. 2h,i and Supplementary Fig. 2d,e ), while seeming to move predominantly by dislodging the matrix. This difference in gelatin invasion was not due to migratory defects, as we found no significant difference between control and VAMP3 shRNA cells migrating on tissue culture glass ( Supplementary Fig. 5 ). Similar results were obtained when control and VAMP3 knockdown cells were plated on pepsin-extracted collagen-I (PurCol). Again, control cells displayed linear paths of invasion, while VAMP3 shRNA cells were visualized as twisting and gyrating, periodically moving laterally only to turn and migrate in the reverse direction. ( Fig. 2j ). When plated on PurCol collagen-I, scrambled control cells invaded an average of 156.8±7.87 μm, while VAMP3 shRNA cells only invaded 26.1±12.11 μm ( Fig. 2k ). Notably, VAMP3 shRNA had no effect on invadopodia degradation characteristically seen in flat, spread cells, while VAMP7 shRNA abolished most invadopodia-mediated degradation at the adherent surface ( Supplementary Fig. 6a–c ). Thus, VAMP3 and VAMP7 have functional roles in matrix degradation at distinct sites TMVs and invadopodia, respectively. VAMP3-CD9 interaction is required for MT1-MMP trafficking The pattern of invasion in VAMP3 knockdown cells was reminiscent of that seen when β 1 -integrin activity was perturbed [32] , [33] . Immunofluorescence using an active integrin antibody (12G10) revealed no difference between control and VAMP3 shRNA cells ( Supplementary Fig. 7 ). Previous reports identified the tetraspanin CD9 as critical for MT1-MMP delivery to the cell surface [34] . Immunoprecipitation of CD9 from both control and VAMP3 knockdown lysates revealed a significant reduction in the amount of co-precipitating MT1-MMP in VAMP3 knockdown cells ( Fig. 3a ). There was no reduction in CD9-β 1 -integrin co-precipitation when VAMP3 was knocked down and no difference in CD9 interaction with the integral endoplasmic reticulum protein BAP-31 as well, which has been linked both to the exit of VAMP3 from the endoplasmic reticulum and the surface expression CD9 (refs 35 , 36 ). We were unable to precipitate this complex using control antibody. The association between tetraspanins and MT1-MMP has been shown to protect the protease from lysosomal degradation [34] . Consistent with these results, we also note, in both melanoma and prostate cell lines, that depletion of VAMP3 leads to an overall decrease in immunostaining for MT1-MMP, suggesting that newly synthesized protease is targeted for degradation rather than surface expression ( Fig. 2f and Supplementary Fig. 4a ). Thus, VAMP3 is required for the association of MT1-MMP with CD9, to enable the routing of MT1-MMP to the plasma membrane. 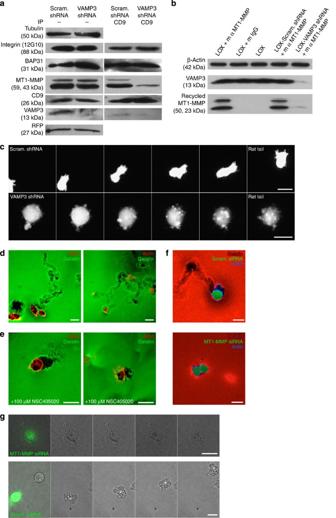Figure 3: VAMP3 depletion disrupts association between MT1-MMP and CD9. (a) Lysates from control-shRNA- or VAMP3-shRNA-electoporated cells were immunoprecipitated using polyclonal anti-CD9 antibody. Total cell lysates (left) and immunoprecipitates (right) were resolved by SDS–PAGE, transferred to polyvinylidene difluoride membrane and probed as indicated. Blots shown are representative of more than four independent immunoprecipitation replicates. (b) LOX cells and those expressing shRNA, as indicated, were incubated with mouse anti-MT1-MMP (lanes 1, 4 and 5) or control mouse IgG (lane 3) as described in Methods. These cells were incubated for 16 h in pre-cleared complete culture media before shed microvesicles were isolated. Microvesicle lysate was then resolved by SDS–PAGE and analysed by western blotting as indicated. (c) LOX cells expressing either scrambled-shRNA or VAMP3-shRNA were embedded in BD Rat Tail collagen I matrix and imaged 24 h post embedding, to allow for shRNA expression. Frames shown are representative stills captured approximately every 20 min. Scale bar, 25 μm. Control (d) or NSC405020-treated (e) LOX cells were plated on FITC-gelatin and allowed to invade overnight. Coverslips were fixed and stained as indicated, to examine the extent of cell invasion. Scale bar, 25 μm. (f) Cells expressing scrambled siRNA (top) or MT1-MMP siRNA (bottom) were allowed to invade TRITC-conjugated matrix overnight. The cells were then fixed, stained as indicated and analysed by confocal microscopy, to examine invasive capacity. Scale bar, 25 μm. (g) LOX cells transfected to express MT1-MMP-siRNA (top) or scrambled siRNA (bottom) were embedded in a layer of rat tail collagen-I and allowed to invade. Cell invasion was monitored by phase-contrast microscopy over the course of 12 h. Stills represent sequential images every 90 min. Scale bar, 25 μm. Figure 3: VAMP3 depletion disrupts association between MT1-MMP and CD9. ( a ) Lysates from control-shRNA- or VAMP3-shRNA-electoporated cells were immunoprecipitated using polyclonal anti-CD9 antibody. Total cell lysates (left) and immunoprecipitates (right) were resolved by SDS–PAGE, transferred to polyvinylidene difluoride membrane and probed as indicated. Blots shown are representative of more than four independent immunoprecipitation replicates. ( b ) LOX cells and those expressing shRNA, as indicated, were incubated with mouse anti-MT1-MMP (lanes 1, 4 and 5) or control mouse IgG (lane 3) as described in Methods. These cells were incubated for 16 h in pre-cleared complete culture media before shed microvesicles were isolated. Microvesicle lysate was then resolved by SDS–PAGE and analysed by western blotting as indicated. ( c ) LOX cells expressing either scrambled-shRNA or VAMP3-shRNA were embedded in BD Rat Tail collagen I matrix and imaged 24 h post embedding, to allow for shRNA expression. Frames shown are representative stills captured approximately every 20 min. Scale bar, 25 μm. Control ( d ) or NSC405020-treated ( e ) LOX cells were plated on FITC-gelatin and allowed to invade overnight. Coverslips were fixed and stained as indicated, to examine the extent of cell invasion. Scale bar, 25 μm. ( f ) Cells expressing scrambled siRNA (top) or MT1-MMP siRNA (bottom) were allowed to invade TRITC-conjugated matrix overnight. The cells were then fixed, stained as indicated and analysed by confocal microscopy, to examine invasive capacity. Scale bar, 25 μm. ( g ) LOX cells transfected to express MT1-MMP-siRNA (top) or scrambled siRNA (bottom) were embedded in a layer of rat tail collagen-I and allowed to invade. Cell invasion was monitored by phase-contrast microscopy over the course of 12 h. Stills represent sequential images every 90 min. Scale bar, 25 μm. Full size image With prior research highlighting the role for VAMP3 in regulating cargo recycling from early endocytic compartments [37] , we sought to determine whether endosomal MT1-MMP, known to be stored intracellularly for rapid delivery to the cell surface [29] , [38] , [39] , was targeted to TMVs and if this inclusion was affected by VAMP3 depletion. Surface MT1-MMP was labelled with anti-MT1-MMP antibody and allowed to internalize. Residual surface antibody was removed and TMVs isolated after 16 h. Western blotting of TMV lysate showed that recycled MT1-MMP is incorporated into shed TMVs and this inclusion is greatly reduced by knocking down VAMP3 ( Fig. 3b ). In addition, VAMP3-positive endosomes, which contain MT1-MMP, also contain ARF6 ( Supplementary Fig. 8 ). These data suggest that VAMP3 is required for the association of MT1-MMP with CD9 and the delivery or recycling of endosomal MT1-MMP to nascent TMVs as well. We speculate that VAMP3 endosomes may be a convergence point for newly synthesized MT1-MMP as well as recycling protease post internalization from the cell surface. Whether CD9 interacts with the protease on endosomes or at the cell surface requires further investigation. Functional TMVs facilitate amoeboid cell invasion High-blebbing rounded cells have been thought to migrate largely by cell propulsion and limited proteolysis [31] . The fact that TMV formation correlates with the spherical and high-bleb phenotype prompted us to address the potential role of TMV-associated proteases in cell invasion. To this end, both scrambled- and VAMP3-shRNA-transfected cells were allowed to invade Rat Tail collagen-I, which still contains telopeptides crucial for cross-linking and fibre formation. An emerging view is that this cross-linking leads to rapid gelling following incubation at physiologic temperatures. Gelling of acid-extracted rat-tail collagen under these conditions results in the formation of a dense fibrillar matrix containing much smaller pores and necessitates proteolytic degradation to allow for cell invasion [40] , [41] . We determined that VAMP3 shRNA-transfected cells were virtually immobile, while control cells were still able to readily invade through the collagen-I matrix ( Fig. 3c and Supplementary Movies 4 and 5 ). The ‘invasive’ capacity of VAMP3 knockdown cells was limited and appeared to be linked to their ability to deform and force themselves through the matrix ( Supplementary Fig. 9 and Supplementary Movie 6 ). These knockdown cells were unable to invade in the same capacity as the control cells, as they lack MT1-MMP-containing TMVs as described above. Consistently, LOX cells treated with the MT1-MMP inhibitor, NSC405020 (refs 42 , 43 ), which specifically inhibits gelatinase activity without inhibiting activation of MMP2, or cells expressing MT1-MMP siRNA ( Supplementary Fig. 10 ) exhibited invasive phenotypes resembling those observed on VAMP3 knockdown in gelatin ( Fig. 3d–f ) and Rat Tail collagen-I ( Fig. 3g ). These studies support the contention that TMVs are important components of the cellular machinery used by tumour cells for movement through dense collagen I microenvironments. Invasive VAMP3-positive TMVs present in ovarian ascites To investigate the physiological and clinical relevance of the TMVs characterized in these studies, we examined for their presence in excess of 30 clinical samples of body fluids. Abdominal ascites, or when ascites was absent, saline wash was collected during exploratory laparoscopy, from fully consented patients with a prior identification of an ovarian mass. Representative nanoparticle tracking analysis of isolated microvesicles showed an enriched population of larger particles relative to unfractionated ascites ( Fig. 4a ). Median particle sizes were 264 and 410 nm in the unfractionated fluid and microvesicle fractions, respectively. Although serous epithelial ovarian cancer was the most common of the cases analysed in this study, samples from patients diagnosed with mucinous, endometroid and clear cell ovarian tumours exhibited similar fractionation profiles. These results were supported by electron microscopy of isolated microvesicle or exosome fractions from patient ascites including those diagnosed with Stage IIB serous adenocarcinoma, IIIC cystadenocarcinoma or mixed epithelial cell carcinoma. Representative images of Stage IIB serous adenocarcinoma microvesicles are shown in Fig. 4b and exosomes in Supplementary Fig. 11 . Isolated TMVs are enriched with VAMP3, MT1-MMP and ARF6, relative to the unfractionated fluid as determined by western blotting ( Fig. 4c ). These TMVs also contain additional cargo molecules that are currently used or being investigated for potential use as biomarkers. One commonly used biomarker for ovarian cancer, and identified on microvesicles, is the glycoprotein cancer antigen 125 (CA-125). CA-125 is significantly enriched in isolated microvesicles ( Fig. 4c ). These microvesicles do not, however, contain elevated levels of human epididymis protein 4, a marker currently undergoing further investigation as a biomarker for use along with CA-125. As we have previously identified functional MT1-MMP as a cargo component in TMVs, we used ascites-derived microvesicles in an in vitro invasion assay. The unfractionated fluid showed areas of broad degradation with TMV and other membrane remnants ( Fig. 4d , left) likely to be due to the presence of soluble proteases within the unfractionated fluid as well as TMV-associated proteases. In contrast, isolated TMVs showed areas of localized proteolytic matrix degradation ( Fig. 4d , right). The invasive capacity of isolated ascites TMVs is dependent on functional MT1-MMP, as incubation of isolated TMVs in the presence of NSC405020 greatly reduced vesicle-associated gelatin degradation ( Fig. 4e ). In addition, serum collected from a subset of patients was also found to contain circulating TMVs that were enriched in ARF6, MT1-MMP, VAMP3 and CA-125, and are also capable of matrix degradation ( Fig. 4f ). 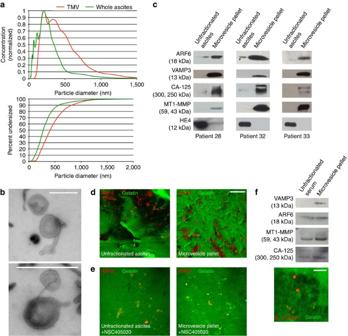Figure 4: Invasive microvesicles can be isolated from peripheral bodily fluids of patients with diagnosed abdomino-pelvic mass. (a) Unfractionated ascites or isolated TMVs were resuspended in sterile, filtered 1 × PBS and subjected to nanoparticle tracking analysis, using a NanoSight LM10 as per the manufacturer’s protocol. Measurements of concentration (upper panel) and percentage undersized (lower panel) versus particle diameter (nm) shown represent the mean of ten individual acquisitions for each sample type. The curves presented are representative of the patient population studied. (b) Microvesicles from patients with Stage IIB serous adenocarcinoma were fixed and examined by whole-mount transmission electron microscopy as described in Methods. Scale bar, 500 nm. (c) Equal amounts of unfractionated ascites fluid and isolated microvesicles (determined using BCA assay) from patient samples were probed by western blotting as indicated.It is worth noting that the protein is equal within but not between patients. Data shown are from patients later diagnosed with serous cystadenocarcinoma of the ovary (28), high-grade serous ovarian carcinoma (32) and poorly differentiated ovarian carcinoma (33). Unfractionated fluid in parallel with isolated TMVs were resuspended in sterile, filtered 1 × PBS (d) or 1 × PBS +NSC405020 (e) before mixing with TMV-free complete cell culture media. The mixture was overlaid onto FITC-gelatin-coated coverslips and allowed to degrade matrix for a period of 14 h. TMVs were fixed, stained as indicated and subjected to confocal microscopy, to examine levels of matrix degradation. Scale bar, 50 μm. (f) Equal amounts of protein from unfractionated serum and isolated TMVs (determined using BCA assay) were probed by western blotting as indicated. In parallel, microvesicles were mixed with 1 × PBS before addition to TMV-free complete cell culture media and incubation with FITC-conjugated gelatin-coated coverslips for a period of 14 h. Scale bar, 10 μm. Data shown are from a patient later diagnosed with serous ovarian carcinoma. Figure 4: Invasive microvesicles can be isolated from peripheral bodily fluids of patients with diagnosed abdomino-pelvic mass. ( a ) Unfractionated ascites or isolated TMVs were resuspended in sterile, filtered 1 × PBS and subjected to nanoparticle tracking analysis, using a NanoSight LM10 as per the manufacturer’s protocol. Measurements of concentration (upper panel) and percentage undersized (lower panel) versus particle diameter (nm) shown represent the mean of ten individual acquisitions for each sample type. The curves presented are representative of the patient population studied. ( b ) Microvesicles from patients with Stage IIB serous adenocarcinoma were fixed and examined by whole-mount transmission electron microscopy as described in Methods. Scale bar, 500 nm. ( c ) Equal amounts of unfractionated ascites fluid and isolated microvesicles (determined using BCA assay) from patient samples were probed by western blotting as indicated.It is worth noting that the protein is equal within but not between patients. Data shown are from patients later diagnosed with serous cystadenocarcinoma of the ovary (28), high-grade serous ovarian carcinoma (32) and poorly differentiated ovarian carcinoma (33). Unfractionated fluid in parallel with isolated TMVs were resuspended in sterile, filtered 1 × PBS ( d ) or 1 × PBS +NSC405020 ( e ) before mixing with TMV-free complete cell culture media. The mixture was overlaid onto FITC-gelatin-coated coverslips and allowed to degrade matrix for a period of 14 h. TMVs were fixed, stained as indicated and subjected to confocal microscopy, to examine levels of matrix degradation. Scale bar, 50 μm. ( f ) Equal amounts of protein from unfractionated serum and isolated TMVs (determined using BCA assay) were probed by western blotting as indicated. In parallel, microvesicles were mixed with 1 × PBS before addition to TMV-free complete cell culture media and incubation with FITC-conjugated gelatin-coated coverslips for a period of 14 h. Scale bar, 10 μm. Data shown are from a patient later diagnosed with serous ovarian carcinoma. Full size image Cell invasion is a multifaceted process relying on the interplay between multiple signalling pathways and processes. The studies described here demonstrate that the v-SNARE VAMP3 directs cargo to nascent TMVs at the cell surface, while VAMP7 directs associated MT1-MMP to distinct sites of invasive activity at invadopodia. These results are compatible with the hypothesis that distinct SNARE protein association serves as a mechanism for cargo sorting and delivery during cell invasion. We suggest that the release of protease-loaded TMVs is the culmination of an intricate cargo sorting and enrichment processes. Although VAMP3-mediated regulation is one mechanism to direct specific cargo to sites of TMV biogenesis, nascent microvesicles at the cell surface may be at the confluence of multiple membrane-trafficking pathways directing specialized cargo to these structures. Indeed, the results presented above suggest that VAMP3- and ARF6-positive recycling endosomes are probably a convergence point for MT1-MMP being recycled to the cell surface and being trafficked to TMVs from the biosynthetic pathway ( Fig. 5 ). 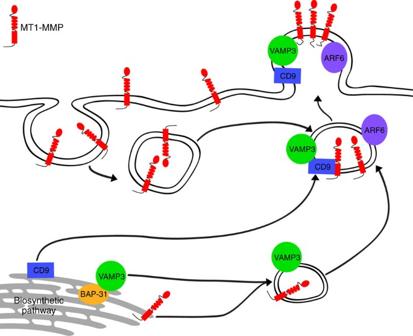Figure 5: Working model for VAMP3-mediated trafficking of MT1-MMP into nascent tumour microvesicles. VAMP3 facilitates interactions between MT1-MMP and CD9, which are required for the routing of newly synthesized MT1-MMP to the cell surface. VAMP3 also regulates the delivery of endosomal MT1-MMP to the cell surface. ARF6- and VAMP3-positive intracellular vesicles may serve as holding and sorting stations for MT1-MMP being delivered to surface TMVs. Whether CD9 interacts with the protease on endosomes or at the cell surface requires further investigation. Figure 5: Working model for VAMP3-mediated trafficking of MT1-MMP into nascent tumour microvesicles. VAMP3 facilitates interactions between MT1-MMP and CD9, which are required for the routing of newly synthesized MT1-MMP to the cell surface. VAMP3 also regulates the delivery of endosomal MT1-MMP to the cell surface. ARF6- and VAMP3-positive intracellular vesicles may serve as holding and sorting stations for MT1-MMP being delivered to surface TMVs. Whether CD9 interacts with the protease on endosomes or at the cell surface requires further investigation. Full size image These studies also demonstrate that proteolytically active TMVs markedly facilitate amoeboid movement and invasion in dense ECM microenvironments. These results are consistent with previous reports that proscribe an essential status to MT1-MMP as a facilitator of cell invasion and ECM proteolysis [44] , [45] , [46] , [47] . We note that the lack of VAMP3 does not limit invasive capacity of rounded cells in all matrix environments. VAMP3-shRNA-expressing cells are still able to invade through softer matrices. It is with denser, more cross-linked matrices such as rat-tail collagen where the invasive defects caused by the loss of endogenous VAMP3 are clearly illustrated. These environments require proteolytic machinery within TMVs to allow for robust invasion as under these conditions; acid-hydrolysed collagen I has previously been documented to form gels containing pores of 1–2 μm diameter [41] . Although we have highlighted the relationship between the shedding of functional TMVs and amoeboid cell invasion, we also note that the molecular mechanisms and/or extracellular cues that may drive cells preferentially towards one mode of invasion over the other remain as fundamental questions in the field. It is unlikely that VAMP3’s role alone, as described here, is driving this transition; however, it could contribute to the mesenchymal-to-amoeboid transition during cell invasion. Future studies examining these relationships will be critical to further understand the complexities of tumour cell invasion. It is reasonable to surmise that the formation and release of proteolytically active microvesicles that can at once prime sites through both paracrine signalling and cell-independent matrix degradation may also greatly enhance the likelihood of metastasis formation. Multiple studies have demonstrated that shed microvesicles are enriched with molecular cargo that is representative of the tumour from which the vesicles originate. This includes not only signatures of the tumour proteome but also detectable levels of both messenger RNA and DNA [1] , [12] . Microvesicle profiles have the potential to be developed into useful diagnostic or prognostic biomarkers for cancers such as ovarian cancer, which currently lack a robust diagnostic tool. As we have demonstrated, ovarian TMVs can be isolated from the peripheral circulation, making them readily accessible for screening—in particlular for tissues such as the ovaries where repeated biopsies to monitor treatment response are impractical. These ovarian TMVs, as we have demonstrated, contain robust and functional MT1-MMP. Knowledge of TMV cargo is of particular importance for ovarian cancers, as they lack a functional anatomical barrier to widespread dissemination. As such, continuing to uncover cargo components sheds additional light on mechanisms of ovarian cancer spread. Furthermore, the fact that disease markers such as CA-125 are contained enriched in the TMV signature relative to the unfractionated fluid provides the added benefit of simultaneous isolation and enrichment of the tumour signature enhancing sensitivity over current techniques. Continuing to uncover cargo trafficking mechanisms and to identify cargo constituents has the potential to radically change the way that we diagnose and treat disease. Antibodies and reagents β 1 -integrin antibody (AIIB2) was obtained from the Developmental Studies Hybridoma Bank at the University of Iowa (1:200); antibodies to β 1 -integrin-12G10 (1:200 immunofluorescence, 1:1,000 western blot), CD9 (1:1,000 western blot, 1:50 immunoprecipitation) and human epididymis protein 4 (1:600) were purchased from Abcam; MT1-MMP antibody was from Millipore (1:100 immunofluorescence, 1:1,000 western blot); anti-RFP antibody was from Rockland Immunochemicals (1:1,200); α-tubulin antibody was obtained from Sigma (1:1,000); antibodies to BAP31 (1:1,000), VAMP3 (1:750) and CA-125 (1:1,000) were purchased from Pierce (Rockford, IL. ); major histocompatibility complex-I antibody was a gift from Dr. Janice Blum (IUPUI, Indianapolis, IN); antibodies to ARF6 were described previously [48] . FITC-phalloidin, AF647-phalloidin, TexasRed and Cy5 secondary antibodies were from Jackson ImmunoResearch (1:300); horseradish peroxidase-conjugated secondary antibodies were purchased from Cell Signaling (1:5,000). GFP-VAMP3 and GFP-VAMP7 were a gift from T. Galli (Institut Jacques Monod, Paris). MT1-MMP-mCherry was a gift from P. Chavrier (Institut Curie, Centre de Recherche, Paris). pRFP-C-RS-VAMP3 shRNA containing sequence 3764 and pRFP-C-RS-scrambled shRNA were purchased from OriGene. Sequence 3764 is 5′- AAACGAGCGAGCCAAGTTGAAGAGGAAA -3′. Cell culture and transfection LOX cell line (provided by Professor Oystein Fodstad, Oslo University) was maintained as previously described [4] . Briefly, cells were cultured in RPMI 1640 (Gibco) supplemented with 10% serum (Hyclone), 2 mM L -glutamine, penicillin and streptomycin. Cultures were maintained at 37 °C and 5% CO 2 in a humidified incubator. PC-3 cells were cultured in F-12K (Gibco) supplemented with 10% serum (Hyclone), 2 mM L -glutamine, penicillin and streptomycin. Transient expression of VAMP3 shRNA plasmids was achieved through transfection using GeneExpresso (Excellgen) (for imaging studies) or electroporation using the NEON electroporation system (for biochemical studies), both according to manufacturer’s protocols. Patient samples Ascites or intraperitoneal saline washings (when ascites was not present) and serum were collected from patients giving informed consent, using the protocol approved by the university’s Human Subjects Institutional Review Boardand the Northern Indiana Cancer Research Consortium Institutional Review Board. Microvesicle isolation Microvesicles and exosomes were isolated by serial centrifugation. Briefly, after 18–24 h, media was removed from actively shedding cells cultured at 60%–75% confluence. Media was centrifuged at 800 g for 10 min and at 2,500i for 15 min, to remove cell debris, and subsequently centrifuged at 10,000 g for 30 min to isolate microvesicles. For patient samples, this 10,000 g pellet was then resuspended in sterile 1 × PBS and centrifuged again at 10,000 g for 30 min. This was repeated for a total of five washes. Isolated vesicles were then used for assays as indicated in text. Additional washes with sterile PBS were conducted on microvesicle pellets from patient samples. Where indicated, exosomes were isolated from microvesicle supernatant by ultracentrifugation at 100,000 g for 60 min. Immunoprecipitations Immunoprecipitations were carried out using co-precipitation buffer (25 mM HEPES, 150 mM NaCl, 5 mM MgCl 2 , 5 mM CaCl 2 , 1% detergent and protease inhibitor cocktail) by lysing cells for 1 h at 4 °C, with gentle rocking. Lysates were cleared and equal amounts of protein incubated with primary antibody for 24 h at 4 °C. Precipitated proteins were then separated by SDS–PAGE and analysed by western blotting. Images have been cropped for presentation with full-size images shown in Supplementary Fig. 12 . Imaging and invasion assays For immunofluorescence, cells or microvesicles were plated on glass, poly- L -lysine- or gelatin-coated coverslips, fixed in 2% paraformaldehyde, washed three times with 1 × X PBS+100 mM glycine, pre-permeabilized with 1 × PBS+0.3% Triton X-100, blocked and permeabilized in 5% BSA, 0.2% Triton X-100, 0.05% Tween-20 in 1 × PBS, and incubated with primary antibodies as indicated in the figures. Following primary incubation, coverslips were washed 3 × followed by incubation with fluorophore-conjugated secondary antibodies and mounted using anti-fade gold mounting media. F-actin distribution was labelled using fluorescently conjugated phalloidin, where indicated. Invasion assays on gelatin or collagen were carried out as previously described, for both cell and microvesicle experiments [4] , [49] . Briefly, cells were trypsinzed and a single-cell suspension overlayed onto coverslips coated with FITC-conjugated porcine skin gelatin. To monitor invasion of isolated microvesicles, the TMV pellet was first resuspended in a small volume of pre-cleared microvesicle-free culture media before being overlayed onto gelatin-coated coverslips. Collagen invasion assays were performed by mixing a single-cell suspension into neutralized collagen-I solution (final concentration, 2 mg ml −1 ), which was then plated on glass bottom dishes and allowed to polymerize at 37 °C. To inhibit endogenous MT1-MMP, NSC405020 (Tocris) was added to cells at 100 μM as previously described [42] , [43] . Immunofluorescence images on fixed cells were acquired using either a Nikon A1R confocal microscope or a BioRad 1024 MRC confocal microscope. Live-cell imaging experiments were conducted using a Nikon spinning disk confocal (× 60 oil-immersion objective or × 20 objective with additional × 1.5 magnification) consisting of a Nikon Ti Eclipse microscope, Yokogawa spinning disk head, CoolSnap HQ camera and environmental control. Systems were controlled using either MetaMorph or iQ2 software. Cells were plated on gelatin substrate for 4 h before imaging. Electron microscopy of isolated microvesicles was carried out as described previously [4] . Briefly, membrane preparations were gently suspended in a small volume of PBS and deposited for 20 min on formvar-carbon-coated electron microscopy grids. The adsorbed membranes were fixed in glutaraldehyde (1%) for 10 min, rinsed with PBS and then with distilled water before contrasting and embedding in a mixture of Uranyl acetate 4%-Methylcellulose 2% (ratio 1:9). All observations were made under a Philips CM120 Transmission Electron Microscope (FEI Company, Eindoven, The Netherlands). Digital acquisitions were generated with a KeenView camera (Soft Imaging System, SIS, Germany). MT1-MMP recycling assay Antibody recycling assays were conducted as described by Park et al . [50] , with anti-MT1-MMP antibody used at 0.2 μg ml −1 . LOX melanoma cells actively shedding TMVs were grown to 60% confluence. These cells were then incubated with 1 × PBS+1% BSA for 20 min at 4 °C, to block nonspecific binding. Blocked cells were then incubated with antibody or IgG control in blocking solution for 120 min at 4 °C. Following antibody labelling, cells were washed once with PBS+100 mM glycine, followed by two washes with cold 1 × PBS. Cells were then gradually warmed to 37 °C in pre-cleared media for 30 min, to allow for internalization of antibody-bound protease. Residual surface antibody was removed by stripping with mildly acidified PBS. Cells were then incubated in pre-cleared media for 16 h, to allow for recycling and TMV shedding. Shed vesicles were collected as previously described [4] and lysates separated by SDS–PAGE. Following transfer to polyvinylidene difluoride membranes were probed with horseradish peroxidase-conjugated anti-mouse antibody to analyse recycled MT1-MMP content in shed TMVs. Western blotting images have been cropped for presentation. Full-size blots are shown in Supplementary Fig. 12 . How to cite this article: Clancy, J. W. et al . Regulated delivery of molecular cargo to invasive tumour-derived microvesicles. Nat. Commun. 6:6919 doi: 10.1038/ncomms7919 (2015).